Experimental proof of nonlocal wavefunction collapse for a single particle using homodyne measurements A single quantum particle can be described by a wavefunction that spreads over arbitrarily large distances; however, it is never detected in two (or more) places. This strange phenomenon is explained in the quantum theory by what Einstein repudiated as ‘spooky action at a distance’: the instantaneous nonlocal collapse of the wavefunction to wherever the particle is detected. Here we demonstrate this single-particle spooky action, with no efficiency loophole, by splitting a single photon between two laboratories and experimentally testing whether the choice of measurement in one laboratory really causes a change in the local quantum state in the other laboratory. To this end, we use homodyne measurements with six different measurement settings and quantitatively verify Einstein’s spooky action by violating an Einstein–Podolsky–Rosen-steering inequality by 0.042±0.006. Our experiment also verifies the entanglement of the split single photon even when one side is untrusted. Einstein never accepted orthodox quantum mechanics because he did not believe that its nonlocal collapse of the wavefunction could be real. When he first made this argument in 1927 (ref. 1 ), he considered just a single particle. The particle’s wavefunction was diffracted through a tiny hole so that it ‘dispersed’ over a large hemispherical area before encountering a screen of that shape covered in photographic film. Since the film only ever registers the particle at one point on the screen, orthodox quantum mechanics must postulate a ‘peculiar mechanism of action at a distance, which prevents the wave... from producing an action in two places on the screen’ [1] . That is, according to the theory, the detection at one point must instantaneously collapse the wavefunction to nothing at all other points. It was only in 2010, nearly a century after Einstein’s original proposal, that a scheme to rigorously test Einstein’s ‘spooky action at a distance’ [2] using a single particle (a photon), as in his original conception, was conceived [3] . In this scheme, Einstein’s 1927 gedankenexperiment is simplified so that the single photon is split into just two wavepackets, one sent to a laboratory supervised by Alice and the other to a distant laboratory supervised by Bob. However, there is a key difference, which enables demonstration of the nonlocal collapse experimentally: rather than simply detecting the presence or absence of the photon, homodyne detection is used. This gives Alice the power to make different measurements, and enables Bob to test (using tomography) whether Alice’s measurement choice affects the way his conditioned state collapses, without having to trust anything outside his own laboratory. The key role of measurement choice by Alice in demonstrating ‘spooky action at a distance’ was introduced in the famous Einstein–Podolsky–Rosen (EPR) paper [4] of 1935. In its most general form [5] , this phenomenon has been called EPR-steering [6] , to acknowledge the contribution and terminology of Schrödinger [7] , who talked of Alice ‘steering’ the state of Bob’s quantum system. From a quantum information perspective, EPR-steering is equivalent to the task of entanglement verification when Bob (and his detectors) can be trusted but Alice (or her detectors) cannot [5] . This is strictly harder than verifying entanglement with both parties trusted [8] , but strictly easier than violating a Bell inequality [9] , where neither party is trusted [8] . To demonstrate EPR-steering quantitatively, it is necessary and sufficient to violate an EPR-steering inequality involving Alice’s and Bob’s results [6] . Such a violation has been shown to be necessary for one-sided device-independent quantum key distribution as well [10] . Because Alice is not trusted in EPR-steering, a rigorous experiment cannot use postselection on Alice’s side [5] , [6] , [11] , [12] , [13] , [14] . Previous experimental tests of nonlocal quantum-state collapse over macroscopic distances, without postselection on Alice’s side, have involved the distribution of entangled states of multiple particles [11] , [12] , [13] , [15] , [16] , [17] , [18] , [19] , [20] , [21] , [22] , [23] , [24] , [25] , [26] , [27] . Experiments demonstrating Bell nonlocality (violating a Bell inequality) for a single photon have involved postselection on both sides, opening the efficiency loophole [28] , [29] ; these lines of work would otherwise have demonstrated EPR-steering of a single photon as well. A recent experimental test of entanglement for a single photon via an entanglement witness has no efficiency loophole [30] ; however, it demonstrates a weaker form on nonlocality than EPR-steering [5] , [6] . While the nonlocal properties of a single particle have spurred much theoretical debate [3] , [31] , [32] , [33] , [34] , [35] , [36] , [37] , [38] , [39] , [40] and many fundamental experiments [28] , [29] , [30] , [41] , [42] , [43] , [44] , [45] , it is also recognized that a single photon split between two spatially distant modes is a very flexible entanglement resource for quantum information tasks: they have been teleported [43] , swapped [44] and purified with linear optics [45] . Spatial-mode entanglement [35] more generally has a broad potential ranging from long-distance quantum communication [46] , [47] , quantum computation [43] , [44] , [45] , [48] , to the simulation of quantum many-body systems in tabletop implementations [49] . In this paper, we rigorously demonstrate Einstein’s elusive ‘spooky action at a distance’ for a single particle without opening the efficiency loophole. We note that, unlike ref. 12 , we do not claim to have closed the separation loophole. Our work is the one-sided device-independent verification of spatial-mode entanglement for a single photon. Our gedankenexperiment First, we explain in detail our simplified version ( Fig. 1 ) of Einstein's original single-particle gedankenexperiment described above, formalized as the task of entanglement verification with only one trusted party, as proposed in ref. 3 . That is, assuming only that Bob can reliably probe the quantum state at his location, he can experimentally prove that the choice of measurement by the distant Alice affects his quantum state. This is exactly the ‘spooky action at a distance’ that Einstein found objectionable [50] . 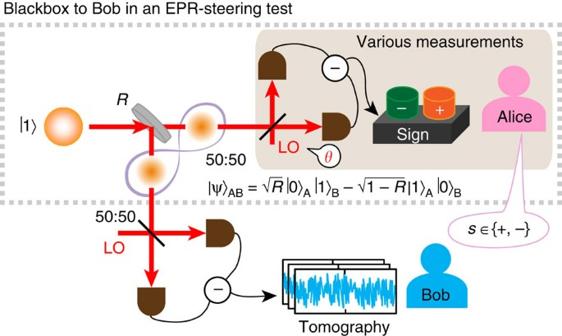Figure 1: Our simplified version of Einstein’s original gedankenexperiment. A single photon is incident on a beam splitter of reflectivityRand then subjected to homodyne measurements at two spatially separated locations. Alice is trying to convince Bob that she can steer his portion of the single photon to different types of local quantum states by performing various measurements on her side. She does this by using different values of her LO phaseθ, and extracting only the signsε{+,−} of the quadrature she measures. Meanwhile, Bob scans his LO and performs full quantum-state tomography to reconstruct his local quantum state. He reconstructs unconditional and conditional local quantum states to test if his portion of the single photon has collapsed to different states according to Alice’s LO settingθ, and results. Figure 1: Our simplified version of Einstein’s original gedankenexperiment. A single photon is incident on a beam splitter of reflectivity R and then subjected to homodyne measurements at two spatially separated locations. Alice is trying to convince Bob that she can steer his portion of the single photon to different types of local quantum states by performing various measurements on her side. She does this by using different values of her LO phase θ , and extracting only the sign s ε{+,−} of the quadrature she measures. Meanwhile, Bob scans his LO and performs full quantum-state tomography to reconstruct his local quantum state. He reconstructs unconditional and conditional local quantum states to test if his portion of the single photon has collapsed to different states according to Alice’s LO setting θ , and result s . Full size image We start with a pure single photon |1› incident on a beam splitter of reflectivity R . As a result, the state of the single photon becomes spread out between two spatially separated modes A and B: The transmitted mode is sent to Alice, and the reflected one to Bob. We allow Alice and Bob to use homodyne detection. This allows Bob to do quantum tomography on his state [51] , [52] , and gives Alice the power to do different types of measurement (which is necessary for an EPR-steering test) by controlling her local oscillator (LO) phase θ . If Alice were simply to detect the presence or absence of a photon, then Bob’s measurement of the same observable will be anticorrelated with Alice's, as in ref. 42 . However, this does not prove that Alice’s measurement affected Bob’s local state because such perfect anticorrelations would also arise from a classical mixture of |0› A |1› B and |1› A |0› B , in which Bob’s measurement simply reveals a pre-existing local state for him, |1› B or |0› B . To demonstrate nonlocal quantum-state collapse, measurement choice by Alice is essential [5] . Following Alice’s homodyne measurement of the θ -quadrature , yielding result , Bob’s local state is collapsed to where the proportionality factor is . Thus, by changing her LO phase θ , Alice controls the relative phase of the vacuum and one photon component of Bob’s conditioned state (modulo π , depending on the sign of the she obtains). Because of this, it is convenient for Alice to coarse-grain her result to . It is possible that a more sensitive EPR-steering inequality could be obtained that makes use of a finer-grained binning of Alices results; however, two bins are sufficient for our experiment. Independently of Alice’s measurement, Bob performs full quantum-state tomography using homodyne detection on his portion of the single photon. This enables him to reconstruct his state, for each value of Alice’s LO setting θ , and coarse-grained result s . Because of the coarse-graining, even under the idealization of the pure state as in Equation (2), Bob’s (normalized) conditioned state will be mixed: The idealized theoretical prediction for the unconditioned quantum state is where P ( s|θ )=0.5 is the relative frequency for Alice to report sign s given setting θ . We once again emphasize the intrinsic lack of trust that Bob has with respect to anything that happens in Alice’s laboratory. Neither her honesty nor the efficiency or accuracy of her measurement devices is assumed in an EPR-steering test. On the other hand, Bob does trust his own measurement devices. From the experimental point of view this means that his photoreceivers do not have to be efficient, and that he can post-select on finding his system in a particular subspace. In particular, for our experiment (where there are small two-photon terms), he can restrict his reconstructed state to the qubit subspace spanned by {|0› B , |1› B }. Despite Bob’s lack of trust in Alice, she can convince him that her choice of measurement setting, θ , steers his quantum state , proving that his system has no local quantum description. We now present data showing this effect qualitatively, before our quantitative proof of EPR-steering for this single-photon system. Bob’s tomography results In our experiment, the (heralded single-photon) input state to the beam splitter comprises mostly a pure single-photon state |1›, but it has some admixture of the vacuum state |0›, and a (much smaller) admixture of the two-photon state |2›. (For more details on state preparation see the Methods.) Following the beam splitter and Alice’s measurement, Bob reconstructs his conditioned quantum states by separately analysing his homodyne data (taken by scanning his LO phase φ from 0 to 2 π ) for each value of Alice’s LO phase θ and result s . The reconstructed density matrices in the {|0› B , |1› B } subspace and the corresponding Wigner functions give complementary ways to visualize how Bob’s local quantum state can collapse in consequence of Alice’s measurement. The results of Bob’s tomography, which take into account inefficiency in Bob’s detection system by using the maximum likelihood method [52] during quantum-state reconstruction, are presented in Fig. 2 , for the case R =0.50. There is good qualitative agreement between these results and the theoretical predictions for the ideal case in Equations (3) and (4). In particular, there are four features to note. 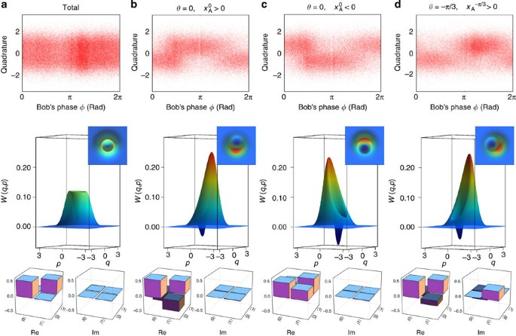Figure 2: Bob’s unconditioned and conditioned quantum states forR=0.50. (a) Bob’s unconditioned data. (b) Bob’s data conditioned onθ=0, positive quadrature sign. (c)θ=0, negative quadrature sign. (d)θ=−π/3, positive quadrature sign. Top: Bob’s marginal distributions (the variation in the number of data points as a function of Bob’s LO phaseφis due to unevenness in Bob’s phase scanning, and does not affect the reconstructions). Middle: reconstruction of Wigner functions (top view in the inset); hereℏ=1 and (q,p) label canonically conjugate quadratures. Bottom: reconstruction of truncated density matrices defined on the {|0›,|1›} subspace; negative elements in darker shade. Figure 2: Bob’s unconditioned and conditioned quantum states for R =0.50. ( a ) Bob’s unconditioned data. ( b ) Bob’s data conditioned on θ =0, positive quadrature sign . ( c ) θ =0, negative quadrature sign . ( d ) θ =− π /3, positive quadrature sign . Top: Bob’s marginal distributions (the variation in the number of data points as a function of Bob’s LO phase φ is due to unevenness in Bob’s phase scanning, and does not affect the reconstructions). Middle: reconstruction of Wigner functions (top view in the inset); here ℏ =1 and ( q , p ) label canonically conjugate quadratures. Bottom: reconstruction of truncated density matrices defined on the {|0›,|1›} subspace; negative elements in darker shade. Full size image First, Bob’s unconditioned quantum state is a phase-independent statistical mixture of the vacuum and single-photon components (see Fig. 2a ), as in Equation (4). The Wigner functions are rotationally invariant, and the off-diagonal terms in are zero. The vacuum component is slightly greater than the single-photon component because of the less-than-unit efficiency p 1 =0.857±0.008<1 of single-photon generation (for more details see the Methods). Second, Bob’s conditioned quantum states are not phase-independent, but rather exhibit coherence between the vacuum and single-photon components (see Fig. 2b–d ) as predicted by Equation (3). The Wigner functions are not rotationally invariant (and have a mean field: ), and the off-diagonal terms in are non-zero. Furthermore, the negative dips observed in the conditioned Wigner functions prove the strong nonclassical character of Bob’s local quantum state [53] . Third, depending on Alice’s result s ε{+,−}, Bob’s local quantum state is collapsed into complementary states (in the sense that they sum to the unconditioned state; compare columns (b) and (c) in Fig. 2 ). This effect is manifested most clearly by a relative π rotation between the conditioned Wigner functions and the opposite signs of the off-diagonal elements of , as expected from Equation (3). Finally, Alice can steer Bob’s possible conditioned states by her choice of measurement setting θ , as predicted. Comparing the results in columns (b) and (d) of Fig. 2 , it is immediately clear that the conditioned Wigner function is phase-shifted with respect to by an angle . Moreover, we also notice the decrease in the value of the real off-diagonal elements and the emergence of the imaginary off-diagonal elements in the conditioned density matrix as compared with . Naturally, the described EPR-steering effect can be demonstrated for all possible values of Alice’s LO phase θ . The above results suggest that Bob’s portion of the single photon cannot have a local quantum state before Alice defining her measurement setting θ . However, a proof that this is the case requires much more quantitative analysis, which we now present. The EPR-steering inequality From Equation (2), Bob’s portion of the single photon is a qubit (a quantum system spanned by |0› B and |1› B ). In the experiment there are small terms with higher photon numbers, but, as explained above, Bob is allowed to restrict to the {|0› B , |1› B } subspace. Here we consider a nonlinear EPR-steering inequality for the qubit subspace. It involves n different measurement settings θ j by Alice, and is given by [3] Here and f ( n ) is a monotonically decreasing positive function of the number of measurement settings defined in Eq. (4.15) of ref. 3 , under the assumption that . The left-hand-side thus correlates Bob’s tomographic reconstruction with Alice’s announced result s , but makes no assumptions about how Alice generates this result. On the right-hand-side, is Bob’s unconditioned state, while . For the ideal case considered above, theory predicts a violation of the EPR-steering inequality (5) for n ≥2 and any value of R (apart from 0 and 1). (However, experimental imperfections associated with the single-photon source and the inefficiency of Alice’s photoreceivers make it more difficult to obtain a violation. For details of the theoretical predictions, see Supplementary Discussion .) While the inequality is most easily violated for n =∞ (for which f (∞)=2/ π ≈0.6366) for our experiment it was sufficient to use n =6 (for which f (6)=0.6440). The experimental results in Fig. 3 well match the theoretical predictions calculated using independently measured experimental parameters; see Supplementary Discussion . The EPR-steering inequality is violated for R =0.08, 0.38 and 0.50, but not for R =0.90; it is most violated at R =0.38 by 0.042±0.006. 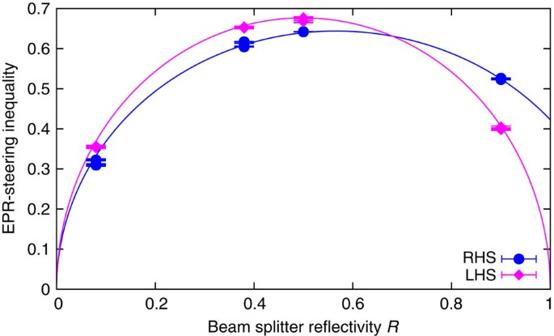Figure 3: The left- and right-hand sides of the EPR-steering inequality. Equation (5) is plotted as a function of the beam splitter reflectivityR. The solid lines show the theoretically predicted values, which take into account the experimental losses, the imperfections associated with the single-photon source and the imperfections of Alice’s homodyne measurements such as phase fluctuations. Four sets of data were taken for eachRto confirm reproducibility of the experimental results. To assess the tomographic errors, error bars were calculated using the bootstrap method, a widely used technique of resampling the data to estimate confidence intervals; for details see ref.55. Figure 3: The left- and right-hand sides of the EPR-steering inequality. Equation (5) is plotted as a function of the beam splitter reflectivity R . The solid lines show the theoretically predicted values, which take into account the experimental losses, the imperfections associated with the single-photon source and the imperfections of Alice’s homodyne measurements such as phase fluctuations. Four sets of data were taken for each R to confirm reproducibility of the experimental results. To assess the tomographic errors, error bars were calculated using the bootstrap method, a widely used technique of resampling the data to estimate confidence intervals; for details see ref. 55 . Full size image The violation of the EPR-steering inequality by seven s.d.’s is a clear proof that Bob’s quantum state cannot exist independently of Alice, but rather is collapsed by Alice’s measurement. We were able to rigorously demonstrate this for a single particle without opening the efficiency loophole by using the combination of multiple ( n =6) measurement settings and highly efficient phase-sensitive homodyne measurements for Alice ( η h =0.96±0.01), coupled with a high single-photon occupation probability ( p 1 =0.857±0.008). Without the close-to-unity values of these parameters, the nonlocal collapse of the single-photon wavefunction could not have been detected, as in the case of ref. 41 (see ref. 3 for a detailed discussion). We have demonstrated, both rigorously and in the easy visualized form of nonclassical Wigner functions, the nonlocality of a single particle using a modern and simplified version of Einstein’s original gedankenexperiment. That is, we demonstrated Einstein’s ‘spooky action at a distance’ in that Bob’s quantum state (of his half of a single photon) was probably dependent on Alice’s choice of measurement (on the other half), and could not have been pre-existing. Quantitatively, we violated a multisetting nonlinear EPR-steering inequality by several s.d.’s (0.042±0.006). This EPR-steering experiment is a form of entanglement verification, for a single-photon mode-entangled state, which does not require Bob to trust Alice’s devices, or her reported outcomes. It was possible only because we used a high-fidelity single-photon state and very high-efficiency homodyne measurements, to perform the steering measurements on Alice’s side and the tomographic state reconstruction on Bob’s. Our results may open a way to new protocols for one-sided device-independent quantum key distribution [10] based on the DLCZ protocol employing single-rail qubits [46] . Experiment Here we present the experimental details of the scheme depicted in Fig. 1 . The source laser is a continuous-wave Ti:sapphire laser of 860 nm. The heralded single photons are conditionally produced based on the set-up presented in ref. 54 at an average count rate of ~8,000 s −1 using a weakly pumped nondegenerate optical parametric oscillator. The single photons are impinged on a beam splitter characterized by reflectivity R , which was set to four different values R ε{0.08,0.38,0.50,0.90}. Alice and Bob perform homodyne measuments on the transmitted and reflected signals, respectively. A piezoelectric transducer is used to control the relative optical path length of the LO of ~10 mW and the signal field, which determines the relative phase. This relative phase is locked, using an Integral (I) feedback control scheme, to one of the six values θ ε{0, ± π /6, ± π /3, π /2} for Alice, and is scanned across the full range [0, 2 π ) for Bob. Overall, 200,000 quadratures, each with an integration time of 500 ns, were recorded for each phase θ , resulting in a total of 1,200,000 quadratures for each data set; the entire experiment took about 20 min for each data set. Four data sets were measured for each beam splitter reflectivity R . Single-photon characterization The experimentally generated heralded single-photon input state to the beam splitter is well modelled by an incoherent mixture of vacuum, single-photon and two-photon contributions given by The input state parameters are p 0 =0.120±0.007, p 1 =0.857±0.008 and p 2 =0.02±0.01 as measured by setting the beam splitter reflectivity to R =1, that is, sending all heralded single photons to Bob, and performing single-mode tomography. The higher-order contributions add up to a negligible value of p h =0.004±0.002. Imperfections of Alice’s measurements The imperfections of Alice’s measurements include the inefficiency and inaccuracy of homodyne detection as well as other losses in Alice’s apparatus. The inefficiency of Alice’s homodyne detection of 1− η h =0.04±0.01 can be attributed to the imperfect spatial mode-match of 0.017±0.004, homodyne detector circuit noise of 0.011±0.002 and the inefficiency of photodiodes (HAMAMASTU, S3759SPL) of 0.01. The inaccuracy of Alice’s homodyne detection is mostly caused by phase fluctuations when locking the relative phase between the signal beam to be measured and the LO: the root-mean-square phase-lock fluctuations are Δ θ =3.9°, estimated from the signal-to-noise ratio of the error signal feedback to the piezo electric transducer used to lock the relative phase to zero. Other losses in Alice’s apparatus are the propagation inefficiency from the optical parametric oscillator to the homodyne detector of 0.015±0.003 and the losses induced by the imperfections of the antireflection coating in the beam splitter, which are 1.07 × 10 −2 ±0.01 × 10 −2 at worst; these add up to an additional loss of l A =0.025±0.007. How to cite this article : Fuwa, M. et al . Experimental proof of nonlocal wavefunction collapse for a single particle using homodyne measurements. Nat. Commun. 6:6665 doi: 10.1038/ncomms7665 (2015).